Superoxide dismutase 1 acts as a nuclear transcription factor to regulate oxidative stress resistance Superoxide dismutase 1 (Sod1) has been known for nearly half a century for catalysis of superoxide to hydrogen peroxide. Here we report a new Sod1 function in oxidative signalling: in response to elevated endogenous and exogenous reactive oxygen species (ROS), Sod1 rapidly relocates into the nucleus, which is important for maintaining genomic stability. Interestingly, H 2 O 2 is sufficient to promote Sod1 nuclear localization, indicating that it is responding to general ROS rather than Sod1 substrate superoxide. ROS signalling is mediated by Mec1/ATM and its effector Dun1/Cds1 kinase, through Dun1 interaction with Sod1 and regulation of Sod1 by phosphorylation at S60, 99. In the nucleus, Sod1 binds to promoters and regulates the expression of oxidative resistance and repair genes. Altogether, our study unravels an unorthodox function of Sod1 as a transcription factor and elucidates the regulatory mechanism for its localization. Reactive oxygen species (ROS) refers to a group of oxygen free radicals that can derive from the environment as a result of radiation or pollutants, or generated as byproducts during normal oxygen metabolic processes such as aerobic respiration in mitochondria or oxidoreductase-catalyzed oxidation. Common ROS include superoxide (O 2 − ) and hydrogen peroxide (H 2 O 2 ) [1] . The superoxide radical is highly reactive but with a very short half life. On the other hand, H 2 O 2 has lower reactivity, which allows the molecule enough time to travel into the nucleus of the cell. Therefore, H 2 O 2 is actually more damaging to DNA than other oxygen free radicals. ROS are reactive with many macromolecules such as lipids, proteins, DNA and RNA, causing their oxidation and loss of normal functions [2] . High ROS level leads to a process that is called ‘oxidative stress’. ROS-dependent oxidation of DNA can generate several different DNA damages, including base modifications, single-strand breaks and intra/interstrand DNA crosslinks [3] . DNA lesions can block progression of replication, causing double-strand breaks. Oxidative damages and the resulting genomic instability are major contributing factors for carcinogenesis. Cellular damages by ROS also play a major role in ageing, diabetic complications, and neurological and cardiovascular diseases. Because of the deleterious effects of ROS, cells have developed sophisticated anti-oxidative system that is continuously processing ROS. The mechanisms for removing ROS involve superoxide dismutases (Sod), catalases, thioredoxin and glutathione [1] . The antioxidants are generally re-cycled to their ‘active’ reduced state by specific enzymes such as glutathione reductase. Sods are a class of highly conserved enzymes that catalyse the dismutation of superoxide into oxygen and H 2 O 2 (ref. 4 ). In eukaryotic cells, there are three distinct superoxide dismutases, Sod1, Sod2 and Sod3. Sod1 is a soluble Cu/Zn enzyme that is mainly in the cytosol, although a small percentage of Sod1 proteins (~3%) were found in the intermembrane space of mitochondria [5] . Sod2 is a manganese enzyme located in the mitochondria, whereas Sod3 is an extracellular enzyme. Sod1 deletion in yeast and mice is known to cause extensive oxidative cellular and genomic DNA damage. Sod1 is known to be a major underlying factor for familial amyotrophic lateral sclerosis, cancer, macular degeneration and muscle atrophy [6] , [7] , [8] , [9] , The past focus of Sod1 has been primarily on the biochemistry of superoxide dismutase enzyme and the disease mechanism of amyotrophic lateral sclerosis. Whether and how Sod1 is regulated under normal and oxidative stress conditions is not well understood. In this study, we show that ATM/Mec1 regulates Sod1 nuclear localization in yeast and humans in response to elevated H 2 O 2 . Inside the nucleus, Sod1 binds to DNA promoters and regulates a programme of gene expression, which is important for resistance to oxidative DNA damage. Oxidative stress promotes Sod1 nuclear translocation To explore possible regulation of Sod1 by oxidative stress, we treated yeast cells with the superoxide-generating agent 4-nitroquinoline-N-oxide (4NQO). Although Sod1 protein level and enzymatic activity ( Fig. 1a ) remain relatively constant, Sod1 localization rapidly changes from predominantly cytoplasmic to prominently nuclear ( Fig. 1b,c ) in a drug dosage-dependent manner ( Supplementary Fig. 1 ). Sod1 nuclear localization also responds to other ROS or ROS-generating agent such as H 2 O 2 , paraquat and menadione ( Fig. 1d,e , Supplementary Figs 2,3 ) but not non-oxidative DNA-damaging or replication stress-inducing chemicals hydroxyurea (HU), methyl methanesulfonate (MMS), zeocin and camptothecan (CPT) ( Fig. 1d,e , Supplementary Fig. 2 ), indicating that Sod1 localization responds to oxidative stress rather than DNA damage. The change in Sod1 localization was verified by subcellular fractionation ( Fig. 1f ). To ask whether Sod1 also responds to changes in endogenous ROS, we analysed Sod1 localization in strains with mutation in GLR1 (glutathione reductase), CTT1 (catalase) or YAP1 (yeast AP-1) that is known to cause elevated ROS [10] ( Fig. 1g ). Compared with WT cells, glr1Δ, ctt1Δ and yap1Δ cells exhibit a marked increase in nuclear Sod1 ( Fig. 1h ), suggesting that endogenous ROS also regulates Sod1 nuclear localization. 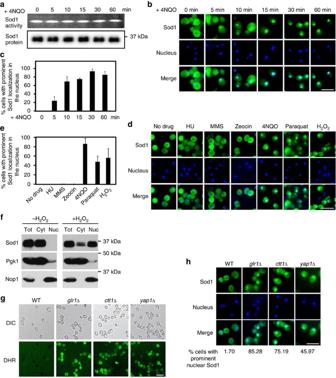Figure 1: ROS induces rapid Sod1 nuclear localization. (a) ROS does not affect Sod1 protein level or enzymatic activity. Yeast cells (SZy1051) were treated with 5 μg ml−14NQO for different times and analysed for Sod1–Myc9 protein level and enzymatic activity. (b) ROS induces rapid nuclear localization. Yeast cells (SZy1051) were treated with 5 μg ml−14NQO for different times and analysed for Sod1–Myc9 localization by IF. The nucleus was stained by DAPI. Scale bar, 10 μm. (c) Shown is the percentage of yeast cells with prominent Sod1 nuclear localization. Error bars indicate ±s.d. of triplicates and at least 100 cells were counted per replicate. (d) ROS but not DNA damageper secauses Sod1 relocalization. Yeast cells (SZy1051) were treated with ROS-generating agents 4NQO, Paraquat or H2O2, or non-oxidative DNA damaging agents HU, MMS and Zeocin and analysed for Sod1–Myc9 localization. Scale bar, 10 μm. (e) Percentage of yeast cells with prominent Sod1 nuclear localization in the experiment depicted in (d). Error bars indicate ±s.d. of triplicates and at least 100 cells were counted per replicate. (f) Sod1 is enriched in the nucleus in response to oxidative stress as determined by subcellular fractionation. Yeast cells were treated without or with 0.4 mM H2O2for 30 min. Yeast cytosol and nuclei were separated by centrifugation and analysed by western blot. Pgk1 and Nop1 were used as cytosolic and nuclear marker, respectively. Tot, total cell extracts; Cyt, cytosol; Nuc, nuclei. (g) Mutation ofGLR1,CTT1andYAP1causes elevated ROS level. Wild type (WT, SZy2492),glr1Δ(SZy2502),ctt1Δ(SZy2503) andyap1Δ(SZy2504) cells under normal culture conditions were stained with dihydrorhodamine (DHR). Scale bar, 10 μm. (h) Increased endogenous ROS is correlated with Sod1 nuclear localization. Sod1–Myc9 localization was analysed by IF in WT (SZy2492),glr1Δ(SZy2502),ctt1Δ(SZy2503) andyap1Δ(SZy2504) cells. Scale bar, 10 μm. Figure 1: ROS induces rapid Sod1 nuclear localization. ( a ) ROS does not affect Sod1 protein level or enzymatic activity. Yeast cells (SZy1051) were treated with 5 μg ml −1 4NQO for different times and analysed for Sod1–Myc9 protein level and enzymatic activity. ( b ) ROS induces rapid nuclear localization. Yeast cells (SZy1051) were treated with 5 μg ml −1 4NQO for different times and analysed for Sod1–Myc9 localization by IF. The nucleus was stained by DAPI. Scale bar, 10 μm. ( c ) Shown is the percentage of yeast cells with prominent Sod1 nuclear localization. Error bars indicate ±s.d. of triplicates and at least 100 cells were counted per replicate. ( d ) ROS but not DNA damage per se causes Sod1 relocalization. Yeast cells (SZy1051) were treated with ROS-generating agents 4NQO, Paraquat or H 2 O 2 , or non-oxidative DNA damaging agents HU, MMS and Zeocin and analysed for Sod1–Myc9 localization. Scale bar, 10 μm. ( e ) Percentage of yeast cells with prominent Sod1 nuclear localization in the experiment depicted in ( d ). Error bars indicate ±s.d. of triplicates and at least 100 cells were counted per replicate. ( f ) Sod1 is enriched in the nucleus in response to oxidative stress as determined by subcellular fractionation. Yeast cells were treated without or with 0.4 mM H 2 O 2 for 30 min. Yeast cytosol and nuclei were separated by centrifugation and analysed by western blot. Pgk1 and Nop1 were used as cytosolic and nuclear marker, respectively. Tot, total cell extracts; Cyt, cytosol; Nuc, nuclei. ( g ) Mutation of GLR1 , CTT1 and YAP1 causes elevated ROS level. Wild type (WT, SZy2492), glr1Δ (SZy2502), ctt1Δ (SZy2503) and yap1Δ (SZy2504) cells under normal culture conditions were stained with dihydrorhodamine (DHR). Scale bar, 10 μm. ( h ) Increased endogenous ROS is correlated with Sod1 nuclear localization. Sod1–Myc9 localization was analysed by IF in WT (SZy2492), glr1Δ (SZy2502), ctt1Δ (SZy2503) and yap1Δ (SZy2504) cells. Scale bar, 10 μm. Full size image Nuclear Sod1 is crucial against oxidative DNA damage To investigate the significance of Sod1 nuclear localization, we generated nuclear and cytoplasmic forms of Sod1 by tagging with an NLS and two different NES peptides that are known to target proteins to the nucleus [11] and cytoplasm [12] , [13] , respectively. As expected, Sod1–NLS and Sod1–NES were localized in the nucleus and cytoplasm, respectively, and their localization did not change by 4NQO treatment ( Fig. 2a ). The superoxide dismutase activity and protein amount of Sod1–NLS and Sod1–NES are similar to WT Sod1 ( Fig. 2b ), indicating different subcellular localizations do not affect Sod1 expression or enzymatic activity. 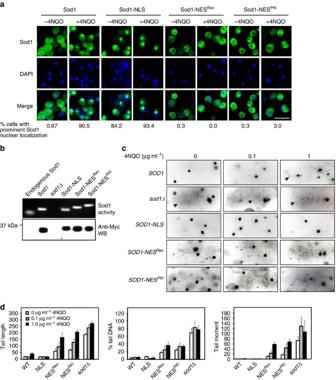Figure 2: Nuclear Sod1 is crucial to protect against genomic DNA damage by ROS. (a) Targeted Sod1 localization in the nucleus or cytoplasm. Yeast cells expressing Sod1–Myc9 (SZy1051), Sod1–NLS–Myc9 (SZy2489), Sod1–NESRev–Myc9 (SZy2499), Sod1–NESPKI–Myc9 (SZy2491) were treated without or with 5 μg ml−14NQO for 30 min, and analysed for Sod1 localization (n>100). Scale bar, 10 μm. (b) Differential subcellular localization does not affect Sod1 protein level or enzymatic activity. The protein level and superoxide dismutase activity of nuclear and cytoplasmic Sod1 were assayed. (c) Nuclear, but not cytoplasmic Sod1 plays a critical role against oxidative DNA damage. Different yeast cells were treated without or with low concentrations of 4NQO for 20 min and assayed for genomic DNA damage by Comet assay. Arrowheads indicate Comet tails. (d) Quantification of the Comet assay results by three different parameters: tail length, % tail DNA and tail moment. Error bars indicate ±s.d. of triplicates and at least 50 cells were counted per replicate. Figure 2: Nuclear Sod1 is crucial to protect against genomic DNA damage by ROS. ( a ) Targeted Sod1 localization in the nucleus or cytoplasm. Yeast cells expressing Sod1–Myc9 (SZy1051), Sod1–NLS–Myc9 (SZy2489), Sod1–NES Rev –Myc9 (SZy2499), Sod1–NES PKI –Myc9 (SZy2491) were treated without or with 5 μg ml −1 4NQO for 30 min, and analysed for Sod1 localization ( n >100). Scale bar, 10 μm. ( b ) Differential subcellular localization does not affect Sod1 protein level or enzymatic activity. The protein level and superoxide dismutase activity of nuclear and cytoplasmic Sod1 were assayed. ( c ) Nuclear, but not cytoplasmic Sod1 plays a critical role against oxidative DNA damage. Different yeast cells were treated without or with low concentrations of 4NQO for 20 min and assayed for genomic DNA damage by Comet assay. Arrowheads indicate Comet tails. ( d ) Quantification of the Comet assay results by three different parameters: tail length, % tail DNA and tail moment. Error bars indicate ±s.d. of triplicates and at least 50 cells were counted per replicate. Full size image Genomic DNA is a major target of oxidative damage. To assess the physiological significance of Sod1 localization, we performed the Comet assay [14] , [15] to measure the level of genomic DNA damage in different yeast strains. Comet tails are barely detectable in untreated WT cells but become visible with 4NQO treatment ( Fig. 2c,d ). Remarkably, Comet tails are already highly prominent in sod1Δ cells even under untreated condition, which are further enhanced in the presence of 4NQO ( Fig. 2c,d ). Essentially, the same DNA damage results were seen with labelling of DNA breaks using the terminal deoxynucleotidyl transferase-mediated dUTP nick-end labelling (TUNEL) assay ( Supplementary Fig. 4 ). Sod1–NES cells behave similarly to sod1Δ cells ( Fig. 2c,d ). In contrast, Sod1–NLS cells resemble WT cells under oxidative stress ( Fig. 2c,d ). Thus, nuclear Sod1 plays a crucial role against genomic DNA damage by endogenous and environmental ROS. ATM/Mec1 regulates Sod1 nuclear localization The dynamic change in Sod1 localization suggests that Sod1 is highly regulated by ROS. ATM kinase is known as an oxidative sensor that is directly activated by H 2 O 2 (ref. 16 ). Additionally, previous work suggested a genetic link between Sod1 and Mec1, a yeast ATM homologue [17] . We hence investigated the role of Mec1 and found that inactivation of the temperature-sensitive mec1-1 allele abrogates the ability of ROS to induce Sod1 nuclear localization ( Fig. 3a ). Intriguingly, yeast proteomic mass spectrometry study revealed that Sod1 forms a potential protein complex with Dun1 (ref. 18 ), a Chk2/Cds1-related protein kinase and a Mec1 effector [19] , [20] . To validate the proteomic result, we affinity-purified Dun1-TAP and found that Sod1 is indeed bound to Dun1 ( Figs 3b , 4a,b ). Furthermore, the Sod1–Dun1 interaction is significantly enhanced by oxidative stress ( Figs 3b , 4a,b ). On other hand, deletion of DUN1 blocks ROS-induction of Sod1 nuclear localization ( Fig. 3c,d ). These observations demonstrate that Dun1 is a bona fide Sod1-binding protein that is required for ROS regulation of Sod1. The fact that Dun1 is a kinase raised the possibility that Sod1 is regulated by phosphorylation. Indeed, two-dimensional (2D) gel detected the appearance of a ROS-induced electrophoretic form of Sod1 protein that is sensitive to phosphatase treatment, indicating that it is a phosphorylated Sod1 ( Fig. 3e , form 3). Moreover, the mec1-1 or dun1Δ mutation abolishes the appearance of this phosphorylated form as a result of 4NQO treatment ( Fig. 3f,g ). Thus, ROS stimulates Sod1 phosphorylation in a Mec1/Dun1-dependent manner. 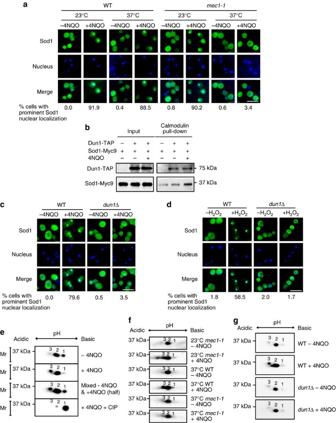Figure 3: ROS-induced Sod1 nuclear localization is dependent on Mec1 and Dun1. (a) Mec1 is required for ROS-induced Sod1 nuclear localization. Exponential WT (SZy2492) andmec1-1(SZy2494) cells at the permissive temperature (23 °C) were maintained at the permissive temperature or switched to the restrictive temperature (37 °C) for 3 h before treated with 5 μg ml−14NQO for 30 min. Sod1–Myc9 localization was then analysed by IF (n>100). Scale bar, 10 μm. (b) ROS stimulates Dun1 interaction with Sod1. Yeast cells expressing Dun1-TAP and/or Sod1–Myc9 (SZy2495, SZy2496, SZy2497) were treated without or with 5 μg ml−14NQO for 30 min. Dun1-TAP was purified by Calmodulin beads. Dun1-TAP and its association with Sod1–Myc9 were analysed. (c) Dun1 is required for 4NQO-induced Sod1 nuclear localization. Exponentially growing WT (SZy2492) anddun1Δ(SZy2493) cells were treated with or without 5 μg ml−14NQO for 30 min, and analysed for Sod1–Myc9 localization by IF (n>100). Scale bar, 10 μm. (d) Dun1 is required for H2O2-induced Sod1 nuclear localization. Exponentially growing WT (SZy2492) anddun1Δ(SZy2493) cells were treated with or without 0.4 mM H2O2for 30 min, and analysed for Sod1–Myc9 localization by IF (n>100). Scale bar, 10 μm. (e) Sod1 is a phosphoprotein and its phosphorylation is stimulated by oxidative stress. Yeast cells (SZy1051) were treated with or without 5 μg ml−14NQO for 30 min. Sod1–Myc9 phosphorylation was analysed by two-dimensional (2D) gel electrophoresis. Different electrophoretic forms are marked by numbers and their status was confirmed by mixing 4NQO-untreated and -treated samples (third panel). (f) Mec1 is required for oxidative stress-induced Sod1 phosphorylation. WT (SZy2492) andmec1-1(SZy2494) yeast cells were cultured at the permissive temperature (23 °C) or restrictive temperature (37 °C) for 3 h before treatment with 5 μg ml−14NQO for 30 min. Sod1–Myc9 was analysed by 2D gel electrophoresis. (g) Dun1 is required for oxidative stress-induced Sod1 phosphorylation. WT (SZy2492) anddun1Δ(SZy2493) yeast cells were treated with 5 μg ml−14NQO for 30 min. Sod1–Myc9 was analysed by 2D gel electrophoresis. Figure 3: ROS-induced Sod1 nuclear localization is dependent on Mec1 and Dun1. ( a ) Mec1 is required for ROS-induced Sod1 nuclear localization. Exponential WT (SZy2492) and mec1-1 (SZy2494) cells at the permissive temperature (23 °C) were maintained at the permissive temperature or switched to the restrictive temperature (37 °C) for 3 h before treated with 5 μg ml −1 4NQO for 30 min. Sod1–Myc9 localization was then analysed by IF ( n >100). Scale bar, 10 μm. ( b ) ROS stimulates Dun1 interaction with Sod1. Yeast cells expressing Dun1-TAP and/or Sod1–Myc9 (SZy2495, SZy2496, SZy2497) were treated without or with 5 μg ml −1 4NQO for 30 min. Dun1-TAP was purified by Calmodulin beads. Dun1-TAP and its association with Sod1–Myc9 were analysed. ( c ) Dun1 is required for 4NQO-induced Sod1 nuclear localization. Exponentially growing WT (SZy2492) and dun1 Δ (SZy2493) cells were treated with or without 5 μg ml −1 4NQO for 30 min, and analysed for Sod1–Myc9 localization by IF ( n >100). Scale bar, 10 μm. ( d ) Dun1 is required for H 2 O 2 -induced Sod1 nuclear localization. Exponentially growing WT (SZy2492) and dun1 Δ (SZy2493) cells were treated with or without 0.4 mM H 2 O 2 for 30 min, and analysed for Sod1–Myc9 localization by IF ( n >100). Scale bar, 10 μm. ( e ) Sod1 is a phosphoprotein and its phosphorylation is stimulated by oxidative stress. Yeast cells (SZy1051) were treated with or without 5 μg ml −1 4NQO for 30 min. Sod1–Myc9 phosphorylation was analysed by two-dimensional (2D) gel electrophoresis. Different electrophoretic forms are marked by numbers and their status was confirmed by mixing 4NQO-untreated and -treated samples (third panel). ( f ) Mec1 is required for oxidative stress-induced Sod1 phosphorylation. WT (SZy2492) and mec1-1 (SZy2494) yeast cells were cultured at the permissive temperature (23 °C) or restrictive temperature (37 °C) for 3 h before treatment with 5 μg ml −1 4NQO for 30 min. Sod1–Myc9 was analysed by 2D gel electrophoresis. ( g ) Dun1 is required for oxidative stress-induced Sod1 phosphorylation. WT (SZy2492) and dun1Δ (SZy2493) yeast cells were treated with 5 μg ml −1 4NQO for 30 min. Sod1–Myc9 was analysed by 2D gel electrophoresis. 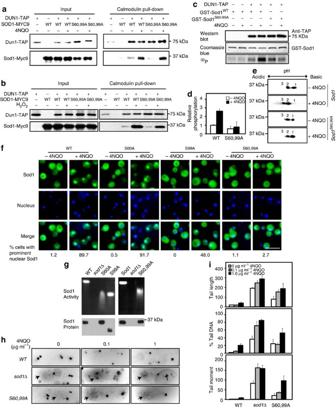Figure 4: ROS stimulates Sod1 phosphorylation at S60 and S99 by Dun1 to promote Sod1 nuclear localization. (a) 4NQO promotes Dun1 interaction with Sod1 and Sod1S60,99A. Yeast cells expressing Dun1-TAP and/or Sod1–Myc9 (SZy2495, SZy2496, SZy2497 and SZy2498) were treated without or with 5 μg ml−14NQO for 30 min. Dun1–TAP interaction with Sod1 proteins were assayed by TAP-pull-down and western blot. (b) H2O2promotes Dun1 interaction with Sod1 and Sod1S60,99A. Yeast cells expressing Dun1–TAP and/or Sod1–Myc9 (SZy2495, SZy2496, SZy2497 and SZy2498) were treated without or with 0.4 mM H2O2for 30 min. Dun1–TAP interaction with Sod1 proteins were assayed. (c) Dun1 phosphorylates Sod1 at S60 and S99 in response to ROS. Yeast cells expressing Dun1–TAP were treated without or with 5 μg ml−14NQO for 30 min. Dun1–TAP was affinity-purified and incubated with bacterial recombinant GST–Sod1 or GST–Sod1S60,99Ain the presence of γ-[32P]-ATP. Phosphorylation of GST-Sod1 proteins was detected by autoradiography. (d) Quantification ofin vitroGST–Sod1 phosphorylation by Dun1–TAP. Error bars indicate ±s.d. of triplicates. (e) The S60, 99A mutations blunt Sod1 phosphorylationin vivo. Exponentially growing yeast cells expressing Sod1–Myc9 or Sod1S60,99A–Myc9 were treated with or without 5 μg ml−14NQO for 30 min. Sod1 phosphorylation was analysed by 2D gel electrophoresis. (f) Phosphorylation at S60 and S99 regulates Sod1 nuclear localization. Yeast cells expressing Sod1–Myc9 (SZy1051), Sod1S60A–Myc9 (SZy2499), Sod1S99A–Myc9 (SZy2500) or Sod1S60,99A–Myc9 (SZy2501) were treated without or with 5 μg ml−14NQO for 30 min. Sod1 localization was analysed by IF. Scale bar, 10 μm. (g) The S60, 99A mutations do not affect Sod1 protein level and enzymatic activity. Yeast cells were cultured under normal conditions. Superoxide dismutase activity (upper panel) and protein expression (Lower panel) were assayed. (h) Sod1S60,99Acells exhibit elevated genomic DNA damage under normal and oxidative stress conditions. Yeast cells expressing Sod1–Myc9 (SZy1051) or Sod1S60,99A–Myc9 (SZy2501) were analysed for genomic DNA damage by the Comet assay in the absence or presence of 4NQO. (i) Quantification of the Comet assay results by three different parameters: tail length, % tail DNA and tail moment. Error bars indicate ±s.d. of triplicates and at least 50 cells were counted per replicate. Full size image Figure 4: ROS stimulates Sod1 phosphorylation at S60 and S99 by Dun1 to promote Sod1 nuclear localization. ( a ) 4NQO promotes Dun1 interaction with Sod1 and Sod1 S60,99A . Yeast cells expressing Dun1-TAP and/or Sod1–Myc9 (SZy2495, SZy2496, SZy2497 and SZy2498) were treated without or with 5 μg ml −1 4NQO for 30 min. Dun1–TAP interaction with Sod1 proteins were assayed by TAP-pull-down and western blot. ( b ) H 2 O 2 promotes Dun1 interaction with Sod1 and Sod1 S60,99A . Yeast cells expressing Dun1–TAP and/or Sod1–Myc9 (SZy2495, SZy2496, SZy2497 and SZy2498) were treated without or with 0.4 mM H 2 O 2 for 30 min. Dun1–TAP interaction with Sod1 proteins were assayed. ( c ) Dun1 phosphorylates Sod1 at S60 and S99 in response to ROS. Yeast cells expressing Dun1–TAP were treated without or with 5 μg ml −1 4NQO for 30 min. Dun1–TAP was affinity-purified and incubated with bacterial recombinant GST–Sod1 or GST–Sod1 S60,99A in the presence of γ-[ 32 P]-ATP. Phosphorylation of GST-Sod1 proteins was detected by autoradiography. ( d ) Quantification of in vitro GST–Sod1 phosphorylation by Dun1–TAP. Error bars indicate ±s.d. of triplicates. ( e ) The S60, 99A mutations blunt Sod1 phosphorylation in vivo . Exponentially growing yeast cells expressing Sod1–Myc9 or Sod1 S60,99A –Myc9 were treated with or without 5 μg ml −1 4NQO for 30 min. Sod1 phosphorylation was analysed by 2D gel electrophoresis. ( f ) Phosphorylation at S60 and S99 regulates Sod1 nuclear localization. Yeast cells expressing Sod1–Myc9 (SZy1051), Sod1 S60A –Myc9 (SZy2499), Sod1 S99A –Myc9 (SZy2500) or Sod1 S60,99A –Myc9 (SZy2501) were treated without or with 5 μg ml −1 4NQO for 30 min. Sod1 localization was analysed by IF. Scale bar, 10 μm. ( g ) The S60, 99A mutations do not affect Sod1 protein level and enzymatic activity. Yeast cells were cultured under normal conditions. Superoxide dismutase activity (upper panel) and protein expression (Lower panel) were assayed. ( h ) Sod1 S60,99A cells exhibit elevated genomic DNA damage under normal and oxidative stress conditions. Yeast cells expressing Sod1–Myc9 (SZy1051) or Sod1 S60,99A –Myc9 (SZy2501) were analysed for genomic DNA damage by the Comet assay in the absence or presence of 4NQO. ( i ) Quantification of the Comet assay results by three different parameters: tail length, % tail DNA and tail moment. Error bars indicate ±s.d. of triplicates and at least 50 cells were counted per replicate. Full size image Dun1 interacts with and phosphorylates Sod1 Several lines of evidence suggested that S60 and S99 of Sod1 are phosphorylated by Dun1. First, recent human phosphoproteomic studies revealed that Sod1 is phosphorylated in both residues [21] , [22] ; second, both residues are conserved between humans and yeast, and S99 was also found to be phosphorylated in a yeast phosphoproteomic study [23] ; third, the 60 S A site of Sod1 is similar to the three Dun1 phosphorylation motifs ( 56 S A 58 S A 60 S S) in Sml1 (ref. 24 ), while AKG 99 S F of Sod1 closely resembles a consensus Dun1 substrate motif (RR X S/T Y ; X , small residues; Y , large hydrophobic residues) as determined by an earlier phosphopeptide display study [25] . To validate S60 and S99 phosphorylation, we mutated these residues to alanine that mimics the un-phosphorylated state. Sod1 S60,99A maintains the ability to bind to Dun1, which is stimulated by treatment with 4NQO or H 2 O 2 ( Fig. 4a,b ). Dun1 phosphorylates bacterially produced GST-Sod1 in vitro , which is enhanced by ROS ( Fig. 4c,d ). However, ROS-induced Sod1 phosphorylation in vitro and in vivo by Dun1 is attenuated by S60, 99A mutations ( Fig. 4c–e ). These results show that these residues are ROS-stimulated Dun1 phosphorylation sites. To address the functional significance of Sod1 phosphorylation, we investigated the effect of Sod1 phosphorylation mutations on Sod1 localization. S60A alone does not significantly affect Sod1 localization. In contrast, S99A partially and S60, 99A completely abrogate ROS-induced Sod1 nuclear localization ( Fig. 4f ). The alanine mutations do not affect Sod1 protein expression or enzymatic activity ( Fig. 4g ). Of note, the mutant proteins do exhibit abnormal electrophoretic mobility on polyacrylamide gels, the nature of which is presently not understood. Sod1 S60,99A cells exhibit increased genomic DNA damage under normal and oxidative conditions ( Fig. 4h,i , Supplementary Fig. 4b ). Collectively, these results show that Dun1 phosphorylates Sod1 at S60 and S99, which regulates Sod1 nuclear localization and is important for genomic stability under normal and oxidative conditions. Nuclear Sod1 regulates gene expression H 2 O 2 is not a substrate of Sod1 and H 2 O 2 burst does not affect cellular superoxide level ( Supplementary Fig. 5 ). Nevertheless, it efficiently stimulates Sod1 nuclear localization ( Fig. 1 ), suggesting that Sod1 nuclear localization is unrelated to catalysing the removal of superoxide. An important cellular defence mechanism against oxidative stress is the induction of genes involved in ROS resistance and DNA damage repair [26] . To address the physiological role of nuclear Sod1, we performed DNA microarray analysis of global gene expression in wild type (WT) and sod1Δ cells before and after treatment with 0.4 mM H 2 O 2 for 20 min. Comparison of the expression profiles of WT ±H 2 O 2 and sod1Δ ±H 2 O 2 revealed 123 genes whose induction by H 2 O 2 was significantly attenuated by SOD1 deletion. Importantly, Sod1-dependent genes fall into five categories that are involved in oxidative responses: oxidative stress, replication stress, DNA damage response, general stress response and Cu/Fe homeostasis ( Fig. 5a–c and Supplementary Fig. 6 ). 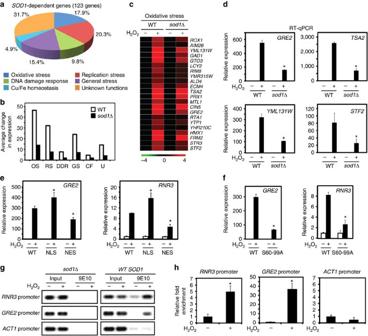Figure 5: Nuclear Sod1 regulates expression of oxidative stress responsive genes. (a) Sod1 is required for the induction of oxidative response (OR) genes. WT orsod1Δ cells were treated without or with 0.4 mM H2O2for 20 min and analysed for global gene expression profile. 123 Sod1-dependent genes were identified and most of the known genes belong to five related functional categories. (b) Shown is the relative induction level of OR genes by H2O2in each category in WT andsod1Δ cells. Data represent average fold change of induction in each category. (c) Shown is the heat map of genes in the oxidative stress response category. (d) Validation of representative genes (GRE2,Genes deRespuesta aEstres 2;TSA2:Thiol-SpecificAntioxidant 2; YML131W;STF2:STabilizingFactor 2) in the oxidative stress response category by RT-qPCR. Error bars indicate ±s.d. from triplicates of two independent experiments. *P<0.05. (e) Nuclear Sod1 is critical for the induction of OR genes. Yeast cells expressing different forms of Sod1 were treated with 0.4 mM H2O2for 20 min. Representative genes were validated by RT-qPCR. Error bars indicate ±s.d. from triplicates of two independent experiments. *P<0.05. (f) The induction of OR genes by ROS was attenuated in Sod1S60,99Acells. Yeast cells expressing Sod1 or Sod1S60,99Awere treated with 0.4 mM H2O2for 20 min. Expression ofGRE2andRNR3were determined by RT-qPCR. Error bars indicate ±s.d. from triplicates of two independent experiments. *P<0.05. (g) ROS treatment increases the association of Sod1 with promoter of oxidative responsive genes. WT (SZy1051) andsod1Δ (SZy1050) cells were treated with 0.4 mM H2O2for 20 min. The binding of Sod1 to representative promoters were analysed by chromatin immunoprecipitation (ChIP). (h) Quantification of the experiment depicted in (g). Error bars indicate ±s.d. from triplicates of two independent experiments. *P<0.05, Student’st-test. Figure 5: Nuclear Sod1 regulates expression of oxidative stress responsive genes. ( a ) Sod1 is required for the induction of oxidative response (OR) genes. WT or sod1 Δ cells were treated without or with 0.4 mM H 2 O 2 for 20 min and analysed for global gene expression profile. 123 Sod1-dependent genes were identified and most of the known genes belong to five related functional categories. ( b ) Shown is the relative induction level of OR genes by H 2 O 2 in each category in WT and sod1 Δ cells. Data represent average fold change of induction in each category. ( c ) Shown is the heat map of genes in the oxidative stress response category. ( d ) Validation of representative genes ( GRE2, G enes de R espuesta a E stres 2; TSA2 : T hiol- S pecific A ntioxidant 2; YML131W; STF2 : ST abilizing F actor 2) in the oxidative stress response category by RT-qPCR. Error bars indicate ±s.d. from triplicates of two independent experiments. * P< 0.05. ( e ) Nuclear Sod1 is critical for the induction of OR genes. Yeast cells expressing different forms of Sod1 were treated with 0.4 mM H 2 O 2 for 20 min. Representative genes were validated by RT-qPCR. Error bars indicate ±s.d. from triplicates of two independent experiments. * P< 0.05. ( f ) The induction of OR genes by ROS was attenuated in Sod1 S60,99A cells. Yeast cells expressing Sod1 or Sod1 S60,99A were treated with 0.4 mM H 2 O 2 for 20 min. Expression of GRE2 and RNR3 were determined by RT-qPCR. Error bars indicate ±s.d. from triplicates of two independent experiments. * P< 0.05. ( g ) ROS treatment increases the association of Sod1 with promoter of oxidative responsive genes. WT (SZy1051) and sod1 Δ (SZy1050) cells were treated with 0.4 mM H 2 O 2 for 20 min. The binding of Sod1 to representative promoters were analysed by chromatin immunoprecipitation (ChIP). ( h ) Quantification of the experiment depicted in ( g ). Error bars indicate ±s.d. from triplicates of two independent experiments. * P< 0.05, Student’s t -test. Full size image Sod1-dependent genes are respectively involved in cellular defence against ROS, ROS-induced DNA replication stress and DNA damage responses, general cellular stress and maintenance of cellular redox state (for simplicity, these genes are collectively called ‘oxidative response’ or OR genes). Selective genes in each category were validated by RT-qPCR ( Fig. 5d , Supplementary Fig. 6b,d,f,h,j ). Moreover, Sod1–NES and Sod1 S60,99A attenuate the induction of OR gene expression ( Fig. 5e,f ), indicating that nuclear Sod1 is important for ROS-induced gene expression. To ask whether Sod1 has a role in transcriptional regulation, we performed chromatin immunoprecipitation (ChIP) and found that ROS treatment increases Sod1 binding to the promoter of RNR3 and GRE2 , but not ACT1 , a control gene that is not regulated by Sod1 ( Fig. 5g,h ). These observations suggest that Sod1 regulates gene expression in response to elevated ROS. Sod1 is the major cytosolic superoxide dismutase responsible for dismutating superoxide, a free radical that is highly reactive and can cause cellular damage. In this study, we found that Sod1 rapidly enters into the nucleus in response to increased level of H 2 O 2 . ROS promotes Sod1 association with the Mec1/ATM effector Dun1/Cds1 kinase and phosphorylation of Sod1 at S60 and S99, leading to Sod1 nuclear localization. H 2 O 2 also stimulates Sod1 nuclear enrichment in human FT169A fibroblasts in an ATM-dependent manner ( Fig. 6a,b ). Moreover, human Sod1 was found to be phosphorylated in S60, 99 in a phosphoproteomic study [21] , [22] . Thus the ATM-dependent regulation of Sod1 nuclear localization by ROS is evolutionarily conserved. H 2 O 2 is known to directly oxidize and activate ATM kinase [16] . In contrast to the very short-lived superoxide free radical, H 2 O 2 has a long half life that allows it to diffuse into the nucleus and cause genomic DNA damage. Together, these observations indicate that H 2 O 2 is the key ROS signal that controls Sod1 nuclear translocation to prevent oxidative genomic damage (see Fig. 6c for a working model). 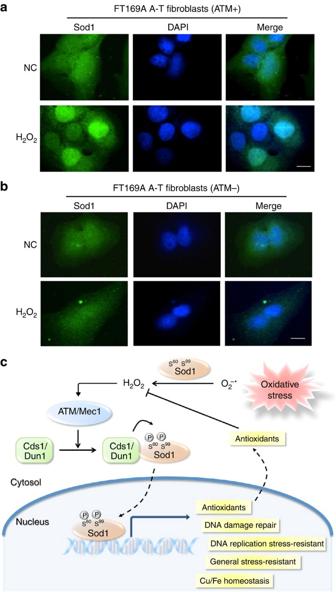Figure 6: ROS rapidly induces Sod1 nuclear localization in human FT169A fibroblasts in an ATM-dependent manner. (a) H2O2burst induces rapid nuclear localization of human Sod1. Human FT169A A-T fibroblasts carrying an ATM-expressing plasmid (ATM+) or a control plasmid (ATM−) were treated with 0.25 mM H2O2for 15 min. Sod1 localization was determined by IF with a human Sod1-specific antibody (green). Nuclear DNA was stained by DAPI (blue). Scale bar, 10 μm. (b) The same as (a) except Human FT169A A-T fibroblasts carrying a control plasmid (ATM−) were used. (c) A working model for Sod1 to act as a nuclear transcription factor to regulate oxidative stress resistance. Figure 6: ROS rapidly induces Sod1 nuclear localization in human FT169A fibroblasts in an ATM-dependent manner. ( a ) H 2 O 2 burst induces rapid nuclear localization of human Sod1. Human FT169A A-T fibroblasts carrying an ATM-expressing plasmid (ATM+) or a control plasmid (ATM−) were treated with 0.25 mM H 2 O 2 for 15 min. Sod1 localization was determined by IF with a human Sod1-specific antibody (green). Nuclear DNA was stained by DAPI (blue). Scale bar, 10 μm. ( b ) The same as ( a ) except Human FT169A A-T fibroblasts carrying a control plasmid (ATM−) were used. ( c ) A working model for Sod1 to act as a nuclear transcription factor to regulate oxidative stress resistance. Full size image The fact that Sod1 is regulated by H 2 O 2 rather than its substrate superoxide, and that H 2 O 2 does not cause an increase in the cellular superoxide level ( Supplementary Fig. 5 ) indicates that the function of nuclear Sod1 is unrelated to the removal of superoxide free radicals. Indeed, we show that nuclear Sod1 regulates the expression of a large set of oxidative response genes that are known to provide resistance to oxidative stress, DNA damage repair and relief of replication stress. For examples, Tsa2 and Prx1 are cytoplasmic and mitochondrial thioredoxin peroxidases, respectively, and are directly involved in the removal of H 2 O 2 ; Rnr3 is the large subunit of ribonucleotide-diphosphate reductase whose expression is important for response to DNA replication stress and DNA damage repair; Rad16, a subunit of nucleotide excision repair factor 4 that is crucial for oxidative DNA damage repair. In addition, a number of Sod1-dependent genes are involved in Fe/Cu homeostasis (for example, Fre1/3/8, iron/copper reductases), which is important for maintaining cellular redox. In response to H 2 O 2 increase, Sod1 becomes associated with the promoters of the target genes, suggesting that Sod1 regulates gene expression at the transcriptional level. Recent evidence also suggested that Sod1 is involved in certain cellular signalling functions. For example, Sod1 was shown to integrate oxygen and glucose signals to repress respiration [27] , though such function involves superoxide and its superoxide dismutase activity. Our study indicates that the well-known enzyme Sod1 that has been studied for nearly half a century has an important new function as a nuclear transcription factor to control general oxidative stress response. As ROS, Sod1 and ATM are broadly involved in normal physiology and diseases, further research in this area could have considerable implications in both basic biology and translational medicine. Chemicals and immunological reagents Oxidative and DNA-damaging drugs HU, MMS, 4-nitroquinoline N-oxide (4NQO), menadione, paraquat and H 2 O 2 were purchased from Sigma-Aldrich. Zeocin was purchased from Invitrogen and CPT was a gift from Dr Leroy Liu of the University of Medicine and Dentistry of New Jersey. Dihydrorhodamine 123 and dihydroethidium were purchased from Life Technology. Mouse anti-Myc (9E10) antibody (#200613) was purchased from Harlan Laboratories. Mouse anti-GST antibody (#2624), anti-mouse horseradish peroxidase (HRP)-conjugated antibody (#7076) and anti-rabbit HRP-conjugated antibody (#7074) were purchased from Cell Signaling Technology. Anti-goat HRP-conjugated antibody (A16142) and Alexa Fluor 488-conjugated goat anti-mouse antibody (A11001) were purchased from Life Technologies. Anti-Sod1 antibody (ab-16831) and anti-PGK1 antibody (ab-113687) were purchased from Abcam. Anti-Nop1 antibody (MCA28F2) was purchased from EnCor Biotechnology. Anti-TAP antibody (CAB1001) was purchased from Thermo Scientific. Protease and phosphatase (PhosSTOP) inhibitor cocktails were purchased from Roche. Yeast strains and plasmids Yeast strains used in this study are listed in Supplementary Table 1 . Mutagenesis of SOD1 was carried out with the QuikChange II Site-Directed Mutagenesis Kit from Agilent Technologies with primers shown in Supplementary Table 2 . SOD1–Myc9 and DUN1–TAP plasmids were constructed by PCR cloning of genomic DNA containing the corresponding tagged ORF and promoter regions into pRS415 and pRS423, respectively [28] . To construct NLS-tagged SOD1 , oligodeoxynucleotide duplex encoding the SV40 NLS sequence (5′-CCTAAGAAGAAGAGGAAGGTT-3′) was inserted into the C terminus of SOD1. To construct NES-tagged SOD1, oligodeoxynucleotide duplex encoding PKI NES (PKI NES ) (5′-TTAGCCTTGAAATTAGCAGGTCTTGATATCAAC-3′) or REV NES (REV NES ) (5′-CTTCAGCTACCACCGCTTGAGAGACTTACTCTT-3′) was inserted into the N terminus of SOD1. GST–SOD1 plasmids were constructed by PCR cloning of SOD1 ORF into pGEX-4T-1 plasmid using the EcoRI and XhoI restriction sites. All plasmid constructs were verified by sequencing and showed proper expression. Drug treatment and indirect immunofluorescence microscopy Exponentially growing yeast cells were treated with oxidative agents 4NQO (5 μg ml −1 ), menadione (0.5 mM), paraquat (1 mM) or H 2 O 2 (0.4 mM) for 1 h, or with DNA-damaging agent HU (100 mM) for 3 h, MMS (0.02%) for 3 h, zeocin (100 μg ml −1 ) for 1 h or CPT (20 μM) for 1 h. The concentration and duration of these drug treatments were used as previously reported [29] , [30] , [31] , [32] , [33] , [34] , [35] . Yeast immunofluorescence studies were performed as described [36] . Anti-Myc (9E10) antibody was used at a dilution of 1:1,000. The antibody–antigen complexes were detected with Alexa Fluor 488-conjugated secondary antibody (1:200 dilution). DNA was stained for 15 min with 50 ng ml −1 4′,6-diamidino-2-phenylindole (DAPI) in antifade mounting medium (Vector Laboratories). Fluorescent images were captured with an Olympus fluorescence microscope equipped with a digital camera. FITC/EGFP/BODIPY filter (Olympus U-N41001) and DAPI/Hoechst/AMCA filter (Olympus U-N31000) were used for detection of the green fluorescence signal of Sod1 and the blue fluorescent signal of nucleus, respectively. Mammalian cell immunofluorescence The immunofluorescence microscopy for mammalian cells was performed as previously described [37] . Briefly, ATM+ or ATM− FT169 A-T fibroblasts obtained from Dr Y. Shiloh, Tel Aviv University, Israel [38] , were grown on coverslips in DMEM (Life Technologies) with 10% FBS (Sigma-Aldrich). After 24 h, the cells were treated with normal media (NC), normal media plus 0.25 mM H 2 O 2 for 15 min, rinsed twice with PBS, fixed with 4% paraformaldehyde and permeated with 0.2% Triton X-100. Cells were blocked with 5% goat serum followed by incubation in anti-human SOD1 primary antibody (1:200 dilution) followed by incubation in Alexa Fluor 488-conjugated secondary antibody (1:200 dilution) and DAPI (Life Technologies) and mounted on microscope slides using CitiFluor mounting media (Ted Pella). Western blot Yeast cells were lysed with glass beads by vortexing in disruption buffer (50 mM Tris-HCl, pH 7.5, 150 mM NaCl, 1 mM EDTA, 1% NP-40, plus protease and phosphatase inhibitor cocktails, Roche). Protein samples were separated by SDS-polyacrylamide gel electrophoresis (PAGE) and then transferred to PVDF membranes. Myc9- and TAP-tagged proteins were detected by anti-Myc (9E10, 1:10,000 dilution) and anti-TAP (1:1,000 dilution) antibodies, respectively. Uncropped images of western blots are shown in Supplementary Fig. 7 . TAP-pull-down assay Yeast cells expressing Dun1-TAP or/and Sod1–Myc9 were cultured to early log phase, and then treated without or with 4NQO for 30 min. Cells were treated with 1% formaldehyde for 30 min to crosslink proteins, followed by incubation in 125 mM glycine for 10 min at 4 °C. Cells were then washed twice with water and resuspended in the pull-down buffer (50 mM Tris-HCl, pH 7.5, 0.5% Triton X-100, 150 mM NaCl, 2 mM CaCl 2 , 5% glycerol, 2 mM PMSF, protease and phosphatase inhibitor cocktails). After cell lysis with glass beads and vortexing, cell lysates were collected by centrifugation at 13,000 rpm and 800 μg total protein in 0.5 ml was incubated with Calmodulin beads (30 μl slurry) for 2 h at 4 °C with rotation. The beads were then washed three times with washing buffer A (50 mM Tris-HCl, pH 7.5, 0.5% Triton X-100, 150 mM NaCl, 2 mM CaCl 2 , 5% glycerol and 2 mM PMSF), once with washing buffer B (50 mM Tris-HCl, pH 7.5, 0.5% Triton X-100, 500 mM NaCl, 2 mM CaCl 2 , 5% glycerol, 2 mM PMSF) and twice with washing buffer C (50 mM Tris-HCl, pH 7.5, 150 mM NaCl, 2 mM CaCl 2 ). The bound materials were eluted from the beads by boiling in SDS protein sample buffer. Dun1–TAP and Sod1–Myc9 were analysed by western blot with anti-Myc (9E10, 1:10,000) and -TAP (1:1,000) antibodies. Sod1 activity assay Yeast cells were washed with phosphate buffer (PB) (0.05 M KH 2 PO 4 and K 2 HPO 4 , pH 7.8) and lysed with glass beads by vortexing in PB supplemented with 0.1% Triton X-100, and protease and phosphatase inhibitor cocktails (Roche). Protein samples (1–5 μg) were separated in 12% native PAGE gel. Sod1 activity assay was carried out as previously described [39] . Briefly, native PAGE gels were stained with 2.43 mM nitro blue tetrazolium chloride (Sigma), 0.14 M riboflavin-5′-phosphate (Sigma) and 28 mM TEMED (Bio-Rad) for 20 min at room temperature in darkness. To visualize Sod1 activity, gels were rinsed with water twice and placed on a light box for 15–120 min. 2D gel electrophoresis Procedure for 2D gel electrophoresis was performed using the ReadyPrep 2-D Starter Kit (Bio-Rad). Briefly, yeast cells were lysed with glass bead by vortexing in 2D sample solubilization solution (8 M urea, 2 mM tributylphosphine (TBP), 4% CHAPS, 0.2% Bio-Lyte Ampholyte (range 4/6), and protease and phosphatase inhibitor cocktails, Roche). Cell extracts were treated with 200 U DNase I (Boehringer Mannheim) for 20 min. Protein samples (1 μg) were diluted in rehydration buffer (sample solubilization solution plus 0.0002% bromophenol Blue), applied to 7-cm immobilized pH gradient (IPG) strips (pH 3.9–5.1), and incubated overnight for sample loading and rehydration. Strips were then isoelectrically focused on a Protein IEF Cell (Bio-Rad) for 14,000 V h. Following isoelectric focusing, the strips were incubated in equilibration buffer I (6 M urea, 2% SDS, 0.05 M Tris-HCl (pH 8.8), 20% glycerol, 2% dithiothreitol) for 10 min. The strips were then incubated with equilibration buffer II (6 M urea, 2% SDS, 0.05 M Tris-HCl (pH 8.8), 20% glycerol, 2.5% iodoacetamide) for 10 min. Second-dimensional separation was performed on 10% SDS-PAGE. Sod1–Myc9 proteins were then transferred to PVDF membranes, and detected by western blot with anti-Myc antibody (1:10,000). For the phosphatase treatment, the cell extract was incubated with calf intestinal phosphatase (20 units, Roche) for 15 min at 30 °C. In vitro kinase assay The in vitro Dun1 kinase assays were performed as described with minor modifications [20] . Briefly, Dun1–TAP was affinity-purified onto Calmodulin-beads and incubated with 20 μCi [γ- 32 P]-ATP in 30 μl kinase buffer (50 mM Tris (pH 7.5), 10 mM MgCl 2 , 60 μM ATP, 1 mM DTT, protease inhibitor cocktail) and 0.1 μg ml −1 purified recombinant bacterial GST–Sod1 proteins for 30 min at 30 °C. Kinase assay was stopped by heating at 100 °C for 5 min in SDS protein sample buffer. The samples were separated on SDS polyacrylamide gels. Protein phosphorylation was detected by autoradiography. Yeast comet and TUNEL assays Yeast comet assay was performed as previously described with slight modifications [40] . Briefly, yeast cells were harvested, resuspended in sorbital buffer (1 M sorbitol, 25 mM KH 2 PO 4 , pH 6.5) and treated with 2 mg ml −1 zymolyase (100T, Seikaguku) for 30 min at 30 °C. Spheroplasts were then washed twice with sorbitol buffer, harvested by centrifugation for 5 min at 2,000 g , and mixed with 1.5% w / v low melting agarose (LMA, type VII, Sigma). This mixture (50 μl) was spread over agarose-coated slide (0.5% w / v LMA, ISC Bioexpress) and immediately covered with a glass cover slip and incubated at 4 °C. After gel solidification, cover slip was removed and 50 μl of LMA was added as the third gel layer. All subsequent steps were performed in cold room at 4 °C. Slides were incubated in yeast comet lysis solution (30 mM NaOH, 1 M NaCl, 0.05% w / v laurylsarcosine, 1% Triton X-100, 50 mM EDTA, 10 mM Tris-HCl, pH 10) for 1.5 h. Slides were then rinsed three times for 20 min in electrophoresis buffer (30 mM NaOH, 10 mM EDTA, 10 mM Tris-HCl, pH 10), followed by electrophoresis in the same buffer for 10 min at 0.75 V cm −1 . After electrophoresis, slides were incubated sequentially in neutralization buffer (10 mM Tris-HCl (pH 7.4)), 75% ethanol and finally 95% ethanol for 10 min each. After air drying, slides were then stained with ethidium bromide (10 μg ml −1 ) for 20 min, rinsed with water for 5 min and covered with glass slip in Vectashield mounting medium (Vector Laboratories). The comet images were captured with an Olympus fluorescence microscope equipped with a digital camera. Comet structural parameters were analysed by the Comet Assay IV software (Perceptive Instruments). For each treatment group, at least 50 comets were analysed and error bars represent s.d. of triplicates. Comet tail length is defined as the length of the comet head diameter subtracted from the overall comet length. Percentage of DNA in the comet tail is defined as the comet tail pixel intensity divided by the total comet pixel intensity, multiplied by 100. The tail moment is computed as the %DNA in the comet tail multiplied by the tail length (Perceptive Instruments). The yeast DNA strand breaks were also determined by the TUNEL assay. TUNEL assay was performed with the In Situ Cell Death Detection kit, POD (Roche Molecular Biochemicals) as described previouly [41] , with minor modification. Briefly, yeast cells were fixed with 3.7% formaldehyde, digested with 300 μg ml −1 Zymolyase 100T and applied to a polylysine-coated slide and allowed to dry for 30 min at 37 °C. The slides were rinsed with PBS, incubated in permeabilization solution (0.1% Triton X-100, 0.1% sodium citrate) for 2 min on ice and rinsed twice with PBS. Slides were subsequently incubated with 10 μl of TUNEL reaction mixture as described in the instruction manual and incubated with diaminobenzidine as a colorimetric substrate. Microscopic images were obtained using an Olympus microscope equipped with a digital camera. Yeast RNA isolation Cells were grown in early log phase (OD 600 ~0.4) when H 2 O 2 was added for a final concentration of 0.4 mM. Samples were collected after 20 min of H 2 O 2 treatment, frozen and stored at −80 °C until RNA extraction. Total RNA was isolated by hot acidic phenol [42] . Briefly, frozen cells were thawed, resuspended in 400 μl of TES solution (10 mM Tris-HCl (pH 7.5), 10 mM EDTA, 0.5% SDS) and incubated with 400 μl of acidic phenol (pH 4.5; Sigma) for 1 h at 65 °C with brief vortexing every 15 min. Samples were placed on ice for 10 min and centrifuged for 5 min at 13,000 r.p.m. at 4 °C. Aqueous (top) phases were extracted with 400 μl phenol as before. Aqueous phases were finally extracted with 400 μl chloroform. RNA was precipitated in 100% ethanol for at least 2 h at −20 °C, centrifuged at 13,000 rpm for 15 min at 4 °C, washed with 70% ethanol and resuspended in H 2 O. Residual DNA was removed by DNase digestion using the RNase-Free DNase Set (Qiagen). RNA samples were further purified by RNeasy Kit (Qiagen). RNA concentration was determined spectrophotometrically by Nanodrop 2000C. Microarray expression profiling and analysis DNA microarray analysis of yeast global gene expression was carried out by Rutgers RUCDR Analytical and Informatics Services using the following procedure. The quality of purified RNA was assessed by Agilent Bioanalyzer 2100 using the Agilent RNA 6000 Nano Kit. RNA concentrations were measured on the Caliper LabChip DS and normalized to 25 ng μl −1 . Samples were amplified and reverse-transcribed using the NuGEN Ovation Pico WTA System V2 with 50 ng RNA according to the manufacturer’s protocol. The yield of resulting cDNA was measured on the Caliper LabChip DS, and product sizing was evaluated on the Bioanalyzer. Five micrograms of each sample were fragmented and labelled with the Nugen Encore Biotin Module following the manufacturer’s protocol. Sizing profiles were assessed once more on the Bioanalyzer to confirm efficient fragmentation (>80% of the material <200 nt in size). Samples were prepared for hybridization to the Affymetrix Yeast Genome 2.0 arrays using the Affymetrix GeneChip Hybridization, Wash and Stain Kit. Modifications were made to the Affymetrix protocol using the cocktail assembly for Mini Arrays. Samples were hybridized overnight in an Affymetrix GeneChip Hybridization Oven 640. Samples were then processed on the GeneChip Fluidics Station 450 and GeneChip Scanner 3000 7G. All arrays were subjected to background correction, normalization and analysis with GeneSifter (Perkin Elmer) software package. Annotations for gene function were mainly derived from the Saccharomyces Genome Database based on the literature [26] , [43] . RT-qPCR Yeast total RNA was reverse-transcribed using gene specific primers and the RETROscript Kit (Ambion) according to the manufacturer’s instruction. The cDNA levels were then analysed using the Rotor-Gene Q 2plex System (Qiagen). Each sample was tested in triplicates using the Rotor-Gene SYBR Green PCR Kit. The primers used for RT and qPCR listed in Supplementary Table 3 were designed using the PrimerQuest programme (Integrated DNA Technologies). To ensure the samples were free from DNA contamination, control samples in which the reverse transcriptase was omitted during cDNA synthesis were run. The thermocycling programme consisted of one hold at 95 °C for 5 min, followed by 40 cycles of 5 s at 95 °C and 10 s at 60 °C. After completion of these cycles, melting-curve data were collected to ensure PCR specificity, contamination and the absence of primer dimers. ACT1 was used for normalization. Relative expression levels were determined by standard curve method [44] . Detection of intracellular ROS and superoxide levels Intracellular ROS and superoxide were detected as described [41] . Briefly, ROS was monitored by staining the cells with 5 μg ml −1 dihydrorhodamine 123 for 2 h with shaking at 30 °C. Cells were then washed with PBS twice and viewed through a fluorescence microscope with a FITC filter (Olympus U-N41001). To monitor intracellular superoxide levels, cells were incubated with 2.5 μg ml −1 dihydroethidium for 10 min with shaking at 30 °C. Cells were then washed with PBS twice and viewed through a fluorescence microscope with a Texas Red filter (Olympus U-N41004). For acquisition of bright-field images, we used an Olympus microscope equipped with a differential interference contrast system. Subcellular fractionation Fractionation of yeast nucleus and cytosol was performed as previously described, with slight modifications [45] . Briefly, yeast cells were spheroplasted with 500 μg ml −1 Zymolyase 100T, homogenized in polyvinylpyrrolidone-buffer (8% polyvinylpyrrolidone, 20 mM potassium phosphate buffer, pH 6.5, 0.75 mM MgCl 2 , and protease and phosphatase inhibitor cocktails) with a Dounce homogenizer. Total lysates were separated by centrifugation (10,000 g for 15 min) into cytosol and nuclei fractions. Sod1–Myc9 and marker proteins for cytosol and nucleus were analysed by SDS-PAGE followed by western blot (9E10, 1:10,000; anti-Nop1, 1:1,000; anti-Pgk, 1:2,000). Chromatin immunoprecipitation (ChIP) Yeast strains were grown to exponential phase, treated with H 2 O 2 for 30 min and fixed with 1% formaldehyde for 30 min. The ChIP assay was performed as described before [46] . For immunoprecipitation, 0.5 mg total protein extracts were incubated with 10 μl of anti-myc (9E10) antibody or control IgG for overnight at 4 °C. Protein-G Sepharose beads were used to recover the antibody–antigen–DNA complexes. The input DNA was prepared in the same way except that the antibody immunoprecipitation steps were omitted. The sod1 Δ strain was used as a control to assess the specificity of the ChIP assay. The primer pairs used for PCR detection are shown in Supplementary Table 3 . Quantification of ChIP results was performed using Quantity One software (Bio-Rad). Accession codes: Microarray data have been deposited in the NCBI Gene Expression Omnibus under accession code GSE55081 . How to cite this article: Tsang, C. K. et al. Superoxide dismutase 1 acts as a nuclear transcription factor to regulate oxidative stress resistance. Nat. Commun. 5:3446 doi: 10.1038/ncomms4446 (2014).